The role of mechanics in biological and bio-inspired systems Natural biological systems are constrained by a limited number of chemical building blocks, yet through practical material organization and mechanics [1] , fulfil the functional needs of diverse organisms by methods that often exceed what is currently achievable using man-made approaches [2] . Synthetic systems are often limited by trade-offs where improving one property comes at the expense of another, as observed when utilizing ceramics in place of metals where a higher elastic modulus is accompanied by lower fracture toughness. However, many natural systems and materials have evolved [3] solutions that result in a number of improved properties simultaneously (for example, high modulus with high fracture toughness), and often produce systems that fulfil multiple functions concurrently. For example, stomatopod dactyl clubs [4] tolerate exceptional amounts of damage through multiphasic material interfaces, and efficient blood-clotting mechanisms are achieved through platelet shape adaptability [5] . These intricate mechanics phenomena, relating material organization and adaptability, are implemented in a structurally minimalistic fashion that is difficult to emulate through artificial manufacturing approaches [6] . Such mechanical functions (that is, mechanofunctionality) of biological systems are not isolated cases—multiscale structural organization also contributes to the hardness of nacre [7] and toughness of toucan beaks [8] , while shape changing commonly drives behaviour in many sea creatures [9] and plants [10] . As such recurrent, mechanically based organizational features throughout biology are discovered and analysed, they provide insight for building exceptional mechanofunctionalities into synthetic, bio-inspired technologies. The survival of organisms is often heightened by structures and materials with favourable properties (for example, load-bearing capacity) or mechanofunctionalities that are passive (without energy input, chemical/mechanical potential only) or active (powered by chemical reactions that transpose to mechanical responses). Such mechanofunctionalities are often based on guiding principles transcending from molecular self-assembly processes to end use. The resulting relationships among mechanics and biology are multi-faceted and circular in the process–structure–function paradigm of engineering. For instance, spiders produce different types of silk through mechanical reeling processes that are tailored for various functions. When building the capture lines of a web, a spider produces stretchy and sticky flagelliform silk. The silk composition and the spinning processes are optimized to form fairly disordered molecular structures that achieve high-extensibility functionality (so-called capture silk) [11] . The spider can alternatively follow a process–structure–function loop to produce dragline silk, which functions as its lifeline during a fall. The rapid reeling during the formation of dragline silk induces mechanical forces that promote the formation of tiny crystalline domains that serve to reinforce the silk and provide greater tensile strength ( Fig. 1a ). 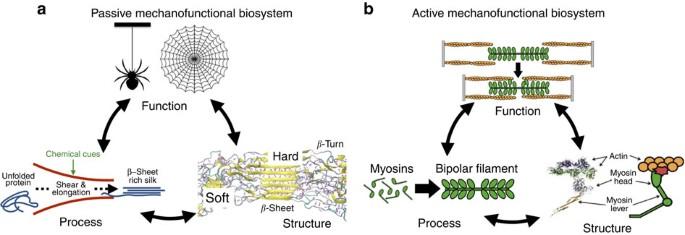Figure 1: Biological systems with passive and active mechanical functions. Process–structure–function. (a) The silk production process of spiders involves the transformation of unfolded proteins into ordered, beta-sheet nanocrystals through shear and elongation. However, not only do chemical factors such as the composition of the solution steer the process, but also mechanical cues such as reeling speed, which changes the shear forces that control polymer chain alignment. These mechanical cues play a fundamental role in the molecular and microscopic structure of spider silk with beta-sheet nanocrystals embedded within amorphous domains. The molecular and microstructural arrangement of the protein building blocks controls mechanical function, whereas the size, orientation and dispersion of beta-sheet nanocrystals and amorphous domains can control strength over extensibility. (b) Filament formation process in muscle systems involves the formation of thick filaments from myosin motor proteins that have globular head and lever/tail domains. Each myosin head extending from the filament acts independently of other heads, while their tail structures intertwine to form the bipolar filament. The molecular configuration of each myosin’s head and lever structure influence their behaviour when cyclically attaching to actin filaments, exerting force and then detaching. In muscles, myosins reaching from bipolar filaments to actin filaments result in contractile muscle functionality. Panelais adapted, with permission, from ref.44(copyright 2015, The Royal Society). Panelbis adapted from refs13and78. Figure 1: Biological systems with passive and active mechanical functions. Process–structure–function. ( a ) The silk production process of spiders involves the transformation of unfolded proteins into ordered, beta-sheet nanocrystals through shear and elongation. However, not only do chemical factors such as the composition of the solution steer the process, but also mechanical cues such as reeling speed, which changes the shear forces that control polymer chain alignment. These mechanical cues play a fundamental role in the molecular and microscopic structure of spider silk with beta-sheet nanocrystals embedded within amorphous domains. The molecular and microstructural arrangement of the protein building blocks controls mechanical function, whereas the size, orientation and dispersion of beta-sheet nanocrystals and amorphous domains can control strength over extensibility. ( b ) Filament formation process in muscle systems involves the formation of thick filaments from myosin motor proteins that have globular head and lever/tail domains. Each myosin head extending from the filament acts independently of other heads, while their tail structures intertwine to form the bipolar filament. The molecular configuration of each myosin’s head and lever structure influence their behaviour when cyclically attaching to actin filaments, exerting force and then detaching. In muscles, myosins reaching from bipolar filaments to actin filaments result in contractile muscle functionality. Panel a is adapted, with permission, from ref. 44 (copyright 2015, The Royal Society). Panel b is adapted from refs 13 and 78 . Full size image In contrast to spider silk, which passively reacts to its environment, active biological systems such as muscle fibres use energy to achieve mechanofunctionality by transducing chemical energy into mechanical energy via myosin motor proteins ( Fig. 1b ). Muscle formation begins with a process of myosin molecules forming bipolar filaments. Myosin isoforms have varied molecular structures that influence their force generation, as well as energy usage rates that inform contractile functionality [12] , [13] . The aggregation of these bipolar filaments into sarcomeres forms the basis of muscles, and the system loops back as environmental feedback from muscle activation influences which myosins are recruited. On the basis of the recruitment of myosins, muscles can achieve fast and powerful contractions or energy-efficient slower contractions. These contrasting examples of spider silk and muscle demonstrate a small subset of the passive and active mechanofunctionalities found in biological systems, where many different strategies have emerged by closing the loop between process and function, while at the same time using mechanics as a key driving force. Such interplays among mechanics and biology are ubiquitous in natural systems. Here we discuss a number of core concepts that have enabled bio-inspired designs and applications to emerge from these approaches. A number of examples explored within this review emphasize systems beyond biomedical applications where mechanics approaches have been traditionally highlighted. We begin at the most fundamental scales by characterizing how natural systems achieve desirable properties using the bottom-up construction of molecular building blocks. A bird’s-eye view is then taken to reveal how emergent system functionality is achieved through multiphase and hierarchical organization across length scales. Finally, we examine the trade-offs among passive and active biological and synthetic materials essential for the design of engineered systems embedded with passive/active mechanofunctionality. With these guiding principles in mind, we then concentrate on different approaches for the design and construction of synthetic biomimetic technologies using core design concepts inspired by nature. Our review aims to provide an informed approach to leverage bio-inspired mechanics-based strategies for integrated mechanical functionality relevant to novel materials, biomedical and nanotechnology applications. Biological systems are primarily constructed through bottom-up self-assembly processes, and the organization of components across length scales informs the mechanics and properties of the system. Despite the limited resources readily available to organisms [14] , many structural materials in biology achieve properties such as ultra-high toughness through clever structuring of a small number of relatively simple carbohydrates, proteins and minerals. Protein-based structural materials, in particular, are unique in their capability to form complex topologies called secondary structures, which arrange hierarchically into larger filaments that serve numerous functions. The impressive properties of protein materials are often directly correlated with the secondary structures of polypeptide repeat units that make up a particular structural material, such as nails and hooves made up of highly crosslinked keratin beta sheets possessing extraordinary hardness [15] . In fibrin and vimentin-like proteins ( Fig. 2a ), alpha-helical folds have repeat units of hydrogen-bonded turns that exhibit large energy dissipation upon unfolding. The reversible energy dissipation and extensibility of these filamentous networks inform structural frameworks with mechanofunctional capabilities of securing blood clots into a scab, and resistance to mechanical perturbations in the cytoskeleton [16] . Other mechanofunctionalities are informed by materials with high elastic energy storage capacity with minimal dissipation, such as resilin and elastin ( Fig. 2b ), where largely disordered, hydrated, networks of biomolecules constitute the nanostructure [17] . Beta-sheet domains in silk ( Fig. 2c ) serve as physical crosslinks that control the outstanding strength of these materials through cooperative hydrogen bonding. These overarching mechanical properties are tied more strongly to structure than sequence, as a number of sequences preserving a few key features can form identical secondary structures that serve as the foundation for embedding targeted mechanofunctions (energy dissipation, extensibility, strength and so on) in synthetic applications. One class of synthetic materials that utilizes these structural features is high-resilience rubber formed from crosslinked resilin [17] , [18] whose molecular and hierarchical structure promotes large energy storage. This material property allows locusts to jump to distances much greater than their size, and enables effective energy storage in the hinges of dragonfly wings. 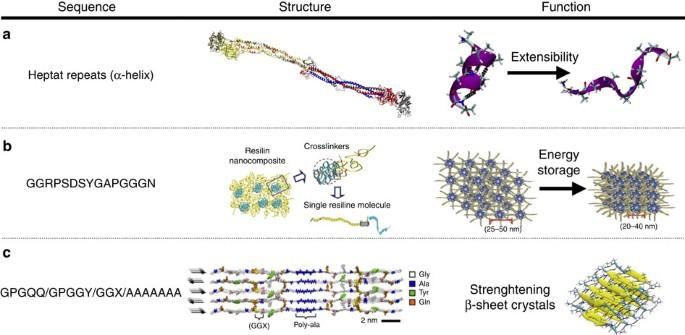Figure 2: Polypeptide repeat units and their mechanical functions. Molecular building blocks consist of biopolymers with repeat sequences that enable the properties of molecular scale structures to scale upwards to observable macroscopic functions. (a) Heptat repeats found in the sequence of proteins including fibrinogen encourage the development of alpha-helices. These alpha-helices promote extensibility when they are unfolded due to an applied force/stress as is observed in the behaviour of blood clots. (b) The sequence of proteins such as resilin promotes the formation of crosslinked nanocomposites that promote energy storage as observed in the hinges of dragonfly wings. (c) Proline–alanine linkages, as observed in spider silk, promote the formation of beta-sheet crystals that are stabilized by hydrogen bonds. Within amorphous domains of spider silk, these beta-sheet crystals serve as reinforcing domains that enhance the strength and stiffness of the material. Together, these three examples help to illustrate the relationship between molecular sequence, structure and function at the nanoscale that ultimately leads to the emergent macroscale properties of natural systems. Panelbis reproduced from ref.17. Panelcis reproduced, with permission, from ref.109(copyright 2015, Elsevier). Figure 2: Polypeptide repeat units and their mechanical functions. Molecular building blocks consist of biopolymers with repeat sequences that enable the properties of molecular scale structures to scale upwards to observable macroscopic functions. ( a ) Heptat repeats found in the sequence of proteins including fibrinogen encourage the development of alpha-helices. These alpha-helices promote extensibility when they are unfolded due to an applied force/stress as is observed in the behaviour of blood clots. ( b ) The sequence of proteins such as resilin promotes the formation of crosslinked nanocomposites that promote energy storage as observed in the hinges of dragonfly wings. ( c ) Proline–alanine linkages, as observed in spider silk, promote the formation of beta-sheet crystals that are stabilized by hydrogen bonds. Within amorphous domains of spider silk, these beta-sheet crystals serve as reinforcing domains that enhance the strength and stiffness of the material. Together, these three examples help to illustrate the relationship between molecular sequence, structure and function at the nanoscale that ultimately leads to the emergent macroscale properties of natural systems. Panel b is reproduced from ref. 17 . Panel c is reproduced, with permission, from ref. 109 (copyright 2015, Elsevier). Full size image Beyond material development, mechanics also affects biological processes at a cellular level, such as force transmitted to the cell nuclei orchestrating the transcription activities that influence embryogenesis [19] and morphogenesis [20] . In these cases, chemical signalling is not enough to fully describe how systems grow, and mechanics have been shown to influence spatiotemporal control of transcriptional activities essential for biological development. There is potential to leverage these principles via engineering approaches, including controlled growth of synthetic biological systems with stretch-activated mechanotransduction for subcellular stimulation via localized mechanical stimulations [21] . Such control would enable techniques of perturbing cells to regulate mechanically guided growth, such as altering localized tissue stiffness that affects neurite outgrowth [22] . Further control could be accomplished through genes that turn on and off in a spatiotemporally controlled manner via macromolecular crowding [23] . Mechanical guidance is especially relevant in stem cell maintenance, differentiation and growth [24] . In these cases, cells can experience force fluctuations attributed to extracellular matrix deformation, internal force changes induced by actomyosin contractility or external forces exerted by neighbouring cells. These forces are then converted internally by the cell into intracellular biochemical signalling (mechanotransduction), which can influence tissue development through cell-to-cell communications, and suggest that engineers could control biological system growth through force perturbations that guide them towards a desirable end state [25] . Such considerations of controlling the growth of biological systems are essential in tissue engineering applications [26] , where many tissue products in the musculoskeletal, cardiovascular and pulmonary systems have mechanical functions for bearing loads, generating force or transporting fluids, and thus require consideration of tuning the growth of a biological system to reach a favourable configuration. Approaches based on mechanics learned from biology can also contribute to understanding and treating cancer, since mechanical force fluctuations throughout a cancer’s microenvironment influence tumorigenesis promotion and metastasis progression [27] . The extracellular matrix, in particular, plays a pivotal role in controlling the microenvironment that influences cancerous growth by regulating the stresses imposed on a tumour [28] . This notion is supported by breast cancer being more common with age as tissues stiffen, which aids disease progression [29] . Evidence of mechanics-based cancer growth has also been demonstrated by confining tumour growth to a small space, which promotes the emergence of leader cells [30] that increase the progression of metastasis. In these cases, the cells have random directionality under no load, but under compression, leader cells have a clear directionality that guides the movement of a group of cells. These mechanics-based findings can aid in developing treatments, and effective approaches could involve mechanical alterations to the cytoskeleton or extracellular matrix, thus ensuring a microenvironment with a distribution of forces that minimizes disease progression. Further research concerning in vivo microenvironment effects on disease progression is essential, and could be supported through in vitro experimental set-ups that closely mimic the physiological conditions of the body [31] . Bottom-up construction of biological systems informs functions beyond the cellular level, and there is the potential for structures to form that are embedded with mechanofunctionality, through specific organizations of molecular units. Many of these systems exhibit extraordinary mechanics in response to environmental stimuli (for example, reversible shape transitions) at a very broad spectrum of spatial (nanometres to metres) and temporal scales (nanoseconds to days) [32] , [33] , [34] , which are a direct result of their make-up at the smallest scales. Passive functionality often emerges from supramolecular biological assemblies with reconfigurable bonds, through which these systems reorganize themselves upon exposure to environmental stimuli; as exemplified by the sorption-induced warping of wood, the curling of hair in hot and humid environments and the slow motions of pinecones, wheat awns and tree branches. Active functionality includes mechanisms such as those of animal muscles, sea organisms or carnivorous plants, where systems utilize energy and generally react faster than passive systems [35] , [36] , [37] . Such functionality that emerges from the system structure can inform the design of man-made functional materials and devices that do more than just serve as structural supports, but also enable mechanical responsiveness to environmental cues for achieving multiple disparate objectives. Features of these passive and active functionalities will be discussed in further detail, but first we present an examination of how designs spanning multiple length scales can also govern a system’s mechanofunctionality. Studying biological system mechanics at the smallest scale does not always provide a complete picture. One exceptional aspect of the biological process is the self-organization of similar biomolecules into disparate phases at the systems level, that is, at greater length scales. Here, we discuss how multiphasic interfaces enhance high-level functionality in biological systems, through highlighted examples including the damage tolerance of the stomatopod dactyl club, the toughness of spider silk and the high strength of cellulose nanocrystals (CNCs). Understanding how multiphasic interfaces and hierarchical organizations across length scales influence emergent macroscale properties in natural systems will aid in developing a materials-by-design approach for novel engineering materials, such as nanocomposites with tailored interfaces and programmed microstructures (for example, the brick-and-mortar arrangement of stiff filler and soft matrix phases observed in nacre [38] ). Despite natural structures utilizing a small catalogue of material components, ingenious organizations significantly bolster their performance beyond that of the pure material components. Such extraordinary properties are demonstrated by the fracture toughness of bone, enamel and dentin, which is several times greater than unstructured hydroxyapatite—the primary mineral found in each material [14] . Beyond structural organization, these building blocks can organize into different phases to achieve superior mechanical properties in many systems. For example, the size and proportion of crystalline and amorphous cellulose phases found in plant cell walls dictate trade-offs between modulus, strength and flexibility, which are foundational for plant survival. Although many of these systems have nanoscale features crucial to macroscale mechanical behaviour, the fine-tuning of material domains across scales is essential and often fulfilled through hierarchical material organizations. One such example is that of nacre’s toughness [7] , attributed to a brick-and-mortar arrangement of stiff, inorganic mineral bricks with soft, organic protein mortar that helps to inhibit crack propagation. Nacre and other hierarchical materials (including bone [39] ) have inspired many materials through biomimetic [2] and materiomics [1] approaches extensively reviewed elsewhere [1] , [2] , [39] . Mimicking such structural and mechanical features in synthetic materials has generated great interest, and man-made multiscale manufacturing approaches in the construction of hybrid multiphasic [6] materials have accelerated the discovery of materials with extreme fracture toughness. In transferring natural system principles to synthetic systems, it is also crucial to recognize that the size of the disparate phases in biological materials requires precise organization beginning at the nanoscale, which is supported by many recent experiments and simulations [40] . One recently discovered and intriguing solution is the stomatopod’s dactyl club that is used to strike highly mineralized prey [4] underwater, therefore requiring exceptional damage tolerance for sustaining instantaneous forces above 500 N. At the microscale, crack propagation via impact is impeded by elastic mismatches of locally parallel chitin fibril stacks with constant skews in angle from the layer below, forming a super-layer with oscillating elastic moduli that is representative of a Bouligand-type structure [41] . On a larger scale, the macroscopic configuration of the club includes three distinct domains: the impact surface, a transitional zone with an abrupt decrease in modulus and hardness with respective values of ∼ 65 and ∼ 3 GPa and a periodic region with oscillating modulus values of 10 and 25 GPa. The combination of multiple phases provides several lines of defence to prevent catastrophic failure during repetitive high-energy loading events. Such clever combinations of material phases across scales are not isolated to stomatopods, or multiscale effects, but emergent mechanofunctionalities can also be attributed to a fine-tuned proportion of materials at a single scale as demonstrated by the impact tolerance of mussel thread networks [42] ( Box 1 ). Mechanical processes involving fields, forces and flows in the environment can also offer structural guidance beyond the chemistry of biological building blocks. Reductionist approaches to understanding the link between molecular repeat units, mechanical properties and relevant mechanical boundary conditions during assembly have facilitated a paradigm shift in identifying design rules in protein materials with mechanofunctions. Such features play a role in making silk tougher than steel [11] , which is attributed to beta-turn and 3 1 -helix-structured amorphous domains combined with hard nanocrystals in its composite nanostructure [43] . This conserved ultrastructure cannot be reproduced by chemistry alone. Mechanical forces arising from elongational shear induced during the spinning process are indispensible driving forces for structural ordering and emergent mechanical properties [44] , [45] . Although environmental features and structural ordering are contributing factors in multiphasic and multiscale materials, nanoscale characteristics of structural building blocks play a similarly important role. New experimental characterization techniques ranging from single-molecule to bulk measurements, as well as computational tools, such as molecular simulations, have greatly enhanced our understanding of mechanofunctionality contained within these building blocks. These studies have gone beyond efforts aimed at identifying the primary sequence of peptides found in structural proteins ( Fig. 2 ) by shedding light on the key role of weak interactions and supramolecular architectures for mechanofunctionality [43] , [44] , [46] , providing key mechanisms of assembly and emergent physical properties. For example, such approaches have aimed to elucidate how hard phases consisting of beta-sheet protein structures found in systems such as amyloid fibrils [16] , nanocrystals in spider silk [16] , [44] , [47] and artificial cyclic peptide nanotubes [48] give rise to outstanding mechanical properties, despite being stabilized by relatively weak hydrogen bonds. One of the most interesting findings to emerge has been the ubiquitous observation that mechanically strong and rigid nanoscale morphologies are formed when small clusters of hydrogen bonds work cooperatively in domains geometrically confined to a few nanometres [46] , [47] , [49] . These results again emphasize the importance of structure and geometry over a specific monomer sequence, as seemingly disparate sequence segments demonstrate nearly identical mechanofunctionality. The multiphasic strategy of spider silk combines a disordered soft phase consisting of noodle-like polymer chain networks that exhibit entropic elasticity, with ordered, hard crystalline phases of beta sheets, where the chains achieve strong alignment. Silk nanocrystals subjected to shear forces break through dissipative stick-slip mechanisms that only emerge when the crystal size is very small, on the order of several nanometres [16] , [44] , [47] . In this case, the sequence of silk couples monomers that easily aggregate into crystalline, beta sheets (alanine) with those that induce extensible, beta turns (most notably proline) and limit the size of these beta-sheet nanocrystals. For silk, sequence and mechanical process govern geometry, which in return governs mechanical properties in a circular fashion ( Fig. 3a,b ). 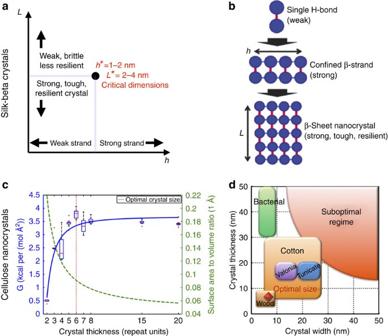Figure 3: Mechanical functions of spider silk and cellulose nanocrystals are influenced by size-dependent effects. (a) The height and length of beta-sheet nanocrystals, such as those found in spider silk, exhibit important critical dimensions (h*andL*) that dictate properties of the macroscale strands including strength, toughness and resiliency. (b) The dimensions of these crystals are confined to a few nanometres to maximize cooperativity of hydrogen bonds, which are individually weak but also cease to work effectively in very large crystals. (c) Cellulose nanocrystals (CNCs) exhibit size-dependent behaviour in the fracture surface energy due to edge defects and scaling of van der Waals interactions between stacked sheets. These crystals have optimal dimensions of 5–7 nm to achieve a robust balance between pull-out failure on the crystal surface (dependent on surface-area-to-volume ratio) and fracture within the crystals (dependent on fracture energy,G). (d) The predicted optimal size of these crystals falls in line with those observed in natural systems and suggests CNCs are nanoscale in size to both maximize fracture toughness and minimize surface to volume ratio. Panelbis reproduced from ref.47. Panelscanddare reprinted, with permission, from ref.50, (copyright 2015, ACS). Figure 3: Mechanical functions of spider silk and cellulose nanocrystals are influenced by size-dependent effects. ( a ) The height and length of beta-sheet nanocrystals, such as those found in spider silk, exhibit important critical dimensions ( h* and L* ) that dictate properties of the macroscale strands including strength, toughness and resiliency. ( b ) The dimensions of these crystals are confined to a few nanometres to maximize cooperativity of hydrogen bonds, which are individually weak but also cease to work effectively in very large crystals. ( c ) Cellulose nanocrystals (CNCs) exhibit size-dependent behaviour in the fracture surface energy due to edge defects and scaling of van der Waals interactions between stacked sheets. These crystals have optimal dimensions of 5–7 nm to achieve a robust balance between pull-out failure on the crystal surface (dependent on surface-area-to-volume ratio) and fracture within the crystals (dependent on fracture energy, G ). ( d ) The predicted optimal size of these crystals falls in line with those observed in natural systems and suggests CNCs are nanoscale in size to both maximize fracture toughness and minimize surface to volume ratio. Panel b is reproduced from ref. 47 . Panels c and d are reprinted, with permission, from ref. 50 , (copyright 2015, ACS). Full size image More recently, a similar size effect was discovered for CNCs [50] that, with an analogous role to the beta sheets in spider silk, are the crystalline reinforcement phase for some of nature’s toughest structural materials, most notably wood. Wood can be thought of as a composite material that combines amorphous and crystalline cellulose, where the amorphous matrix provides flexibility and CNCs, despite their small size, provide significant strength, stiffness and toughness. To help explain this small size of CNCs observed in natural systems, molecular simulations were conducted and have shown that the energy required to fracture a single CNC reaches an asymptotic value at a relatively short length scale of a few nanometres ( Fig. 3c ) [50] . However, the size of these crystals within composites such as wood must also maximize the surface-area-to-volume ratio to prevent failure at interfaces of amorphous and crystalline domains. The ideal size predicted from simulation is in good agreement with the observed size in natural systems ( Fig. 3d ) [50] , suggesting that their size is optimized to resist both interfacial failure and crystal breaking. These results are also relevant to the development of synthetic polymer–CNC nanocomposites, as they provide guidance towards choosing an appropriate size CNC to use as filler material to optimize performance. On the basis of these diverse examples, it is clear that factors such as mechanical size effects, structural/multiscale organizations, interfaces between disparate phases and environmental driving factors greatly influence the behaviour and properties of natural systems. Continued progress towards understanding and characterizing these phenomena will ultimately provide new strategies and tools to incorporate into the design of synthetic materials with inherent mechanofunctionality. Box 1: Dynamic loading response of mussel threads. Evolutionary processes can form intriguing mechanical solutions that enable organisms to thrive in harsh environments, as demonstrated by Mytilidae marine mussels that survive repeated forces from ocean waves [42] . The impact tolerance achieved by marine mussels is non-obvious; tests demonstrate that mussel threads fail at ∼ 5 N, which is much lower than the high-impact dynamic loads of 25 N experienced at sea. However, mussels at sea do not fail. Computational simulations reveal that an emergent functionality among hard and soft materials in mussel threads provides a mechanofunctional dynamic response essential for their survival [41] . The interaction among these materials leads to an initial linear regime of force extension, governed by soft proximal portions of each mussel filament, followed by a stiffening regime where both proximal and distal portions of filaments contribute. Further simulations demonstrated that the maximum impact force for the mussel system is about 48.5 N, which is nearly 10 times greater than the network’s static strength. These results contradict prevalent theories that mussels remain attached due to robust strength in their adhesive plaque structures (see below figure), which have inspired biomimetic approaches for designing antibacterial hydrogels and tissue adhesives with similar functionality [51] . In contrast, these new findings can serve to inform bio-inspired dynamic loading designs based on clever material distribution that overcome trade-offs among energy dissipation and deformation, such as earthquake-resistant structures. Further investigations suggest that the 80:20 distribution of materials in the mussel thread are an optimal ratio for achieving such functionality, and the correct proportion of materials can affect the performance of a design as much as proper material selection. The figure is adapted from ref. 42 . Understanding the role of mechanics in biology provides a number of key evolutionary design principles, but perhaps an even greater consequence is that this knowledge can be further transferred to engineered systems that can mimic and/or surpass the performance of natural systems. Recent efforts in realizing synthetic bio-based technologies have led to many successes in mimicking passive material properties that require no energy expenditures, such as adhesion [51] , elasticity [17] , strength and toughness [52] , self-healing [53] and stimuli responsiveness [54] . In addition, many active, biomimetic systems that do utilize energy to carry out their mechanical functions have also been produced, including synthetic bio-actuators [55] , contractile polymers [56] and electrospun climbing fibres [56] . To facilitate the development of future engineering applications, there is a need to classify and assess the trade-offs among synthetic and biological materials, which achieve useful mechanical functions. Here, we concentrate specifically on passive and active actuation mechanisms, and present a categorization of mechanofunctional materials and systems according to their actuation time and force capabilities ( Fig. 4 ) [9] , [57] , [58] , [59] , [60] , [61] , [62] , [63] , [64] , [65] , [66] , [67] , [68] , [69] . These systems span many orders of magnitude and illustrate a significant breadth of biological and synthetic capabilities to operate in diverse mechanical environments. 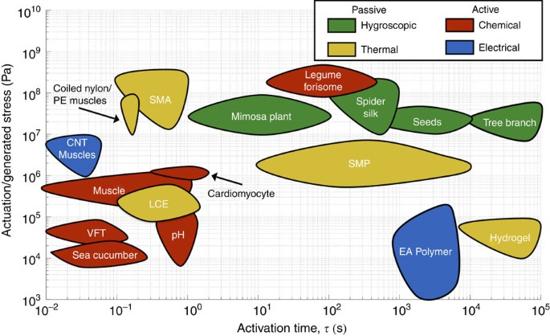Figure 4: ‘Ashby-like’ plot comparing dynamic actuation properties of biological and engineered systems. Systems are classified according to their actuation/generated stress (defined as the stress generated when the material/system undergoes some defined actuation such as muscle contraction or seed opening) and their activation time (time required to complete an actuation cycle). Systems are further classified by colour in terms of the mechanism of their activation and include chemical (red) and electrical (blue) active mechanisms, as well as hygroscopic (green) and thermal (yellow) passive mechanisms. The specific systems included in this figure (abbreviations used in the figure are shown in parentheses) are the sea cucumber dermis9, venus fly trap (VFT)69, human muscle contraction59, pH-activated polymers (pH)59, liquid crystal elastomers (LCE)99, shape-memory alloys (SMAs)63, mimosa plant64, legume forisomes62, shape-memory polymers (SMPs)67, electroactive polymers (EAPs)59, tree branch movement57, seed opening110, carbon nanotube (CNT) muscles65, electrically activiated hydrogels61,66, coiled nylon and polyethylene (PE) muscles60, cardiomyocytes68and spider silk58. Figure 4: ‘Ashby-like’ plot comparing dynamic actuation properties of biological and engineered systems. Systems are classified according to their actuation/generated stress (defined as the stress generated when the material/system undergoes some defined actuation such as muscle contraction or seed opening) and their activation time (time required to complete an actuation cycle). Systems are further classified by colour in terms of the mechanism of their activation and include chemical (red) and electrical (blue) active mechanisms, as well as hygroscopic (green) and thermal (yellow) passive mechanisms. The specific systems included in this figure (abbreviations used in the figure are shown in parentheses) are the sea cucumber dermis [9] , venus fly trap (VFT) [69] , human muscle contraction [59] , pH-activated polymers (pH) [59] , liquid crystal elastomers (LCE) [99] , shape-memory alloys (SMAs) [63] , mimosa plant [64] , legume forisomes [62] , shape-memory polymers (SMPs) [67] , electroactive polymers (EAPs) [59] , tree branch movement [57] , seed opening [110] , carbon nanotube (CNT) muscles [65] , electrically activiated hydrogels [61] , [66] , coiled nylon and polyethylene (PE) muscles [60] , cardiomyocytes [68] and spider silk [58] . Full size image A significant portion of the actuation mechanisms presented in Fig. 4 are plant based [57] , [62] , [64] , [69] , including seed opening, the movement of tree branches and mechanical predatory responses (Mimosa plant and Venus flytrap). The behaviour of these plant-based actuators vary considerably from slow hygrothermomechanical mechanisms that respond to changes in chemical potentials [57] , such as environmental moisture content, to the faster Mimosa plant [64] and legume forisome [62] mechanisms and to the incredibly rapid and high-force actuations of the Venus flytrap [69] activated by chemical stimuli. Such quick actuations in the flytrap are achieved on the order of microseconds via electrochemically activated processes involving motor cells that leverage structural instabilities triggered by turgor pressure. Although they serve drastically different purposes, muscles in animals operate on similar principles, and utilize chemical energy for their varied contractile responses [59] , [68] . Trade-offs also exist among man-made shape-memory polymers and alloys that have passive actuation properties in response to temperature and moisture [63] , [67] . These materials typically operate over a fairly narrow stimulus range, but pH, electroactive polymers and light-activated materials can expand the spectrum of dynamic capabilities for synthetic designs. When comparing all types of materials simultaneously in Fig. 4 , it is clear that there are many potential strategies to optimize systems with mechanofunctionality using different stimuli and environmental cues. It is important to consider a range of actuation candidates in synthetic design applications, since no single material will meet the functional needs of all applications or optimal performance. For instance, passive actuation systems inspired by nature are finding new applications in biomaterials, where electrochemically driven active systems are limited by stability/compatibility issues and the need for basic stimuli/energy for activation. These limitations are addressed by hygrothermomechanical actuators that passively use structural anisotropy [10] to undergo structural transformations under the influence of external changes in moisture and temperature. Contrary to synthetic shape-changing materials such as shape-memory alloys or shape-memory polymers that rely on specific material chemistries, structural anisotropy is more easily developed as it simply involves a specific material organization. Such organization in plants ranges from the anisotropic nano- and microstructures within the cell wall to macroscopic seed dispersal units (that is, wheat awns, pinecones, fern spores and so on) that are activated by external water stimuli [70] . These actuation processes are driven by the static orientation of cellulose fibrils that heavily influence the directional swelling of plant cells, causing actuation of the system over a range of timescales from seconds to days [71] . A number of synthetic materials have been produced that mimic these programmed microstructures and allow for shape [56] or stiffness [54] changes in response to external stimulus. However, the advantages offered by passive, hygrothermal activation mechanisms are counteracted by slower activation time where chemically or electrically driven mechanisms possess an advantage. This specific comparison illustrates the clear trade-offs between different actuation mechanisms that must be considered in designing new, functional materials. Among the many trade-offs in materials for implementing mechanical biomimetic functionality, manufacturing concerns are paramount, and there are many feasible routes of recreating mechanofunctionality in biomimetic systems. In muscle-based systems [60] , [72] , actuation is achievable through biological, synthetic or combinations of both manufacturing approaches—the route chosen plays a pivotal role in the capabilities and trade-offs engineers may vary to meet performance requirements ( Box 2 ). Tissue engineering approaches for synthetic biological muscle could enable design and manufacturing of tissues from the bottom-up [73] , and may eventually offer many options in calibrating a muscle response through altering their myosin motor protein content with synthetic myosins tailored for a specific functionality [13] , [74] . There is a strong correlation between muscle contraction speed and energy consumption to its myosin isoform composition [12] , [75] , which makes these molecules a key consideration in designing muscle tissues. Myosin isoforms vary considerably in nature [76] , [77] and operate via a swinging lever arm domain that governs their mechanical actions, and a head domain responsible for their binding kinetics with actin and adenosine triphosphate. Both the lever and head domains may be tuned synthetically through altering amino-acid sequences or building chimeras from combinations of myosins [74] , [78] . There is great potential in using these myosin engineering and manufacturing techniques in formalizing design approaches [13] , [79] to construct biomimetic devices, such as smart contractile materials, molecular sensors and nano-actuators with optimized responses. These muscle and myosin-based approaches fit into a more general scheme of synthetic biological manufacturing processes that include (i) recombinant approaches for generating mixtures of biomolecules synthesized through genetically engineered bacteria, (ii) hybrid approaches for integrating biomolecules with synthetic materials such as polymers and (iii) biomimetic approaches for developing synthetic materials that directly mimic the mechanofunctionality of natural systems. The first bio-inspired design approach involves reproducing or reengineering assembly processes of biological components produced via recombinant synthesis. Elastomeric protein-based biomaterials are one such example in which elastic proteins (that is, elastin, resilin and so on) can be assembled into various forms (hydrogels, films and scaffolds) or further combined with a synthetic polymer to form new biomaterials [17] , [80] , [81] . In these recombinant approaches, the inherent properties of biomolecules are used in applications that can vary significantly from those observed in nature. For example, these elastic proteins are typically found in the hinges of dragonfly wings, but are used in practical applications simply to exploit the energy storage capabilities of the materials, and are often used in unrelated fields such as medicine/tissue engineering in the development of artificial vocal chords and tissue grafts [81] . Beyond recombinant approaches [54] , incorporating building blocks extracted from natural biosynthesis processes into engineered polymers can give rise to hybrid materials with novel functions. These hybrid approaches aim to incorporate mechanofunctionality, observed in biomolecular blocks, directly into engineered polymer systems by utilizing the efficiency and precise nanomanufacturing capabilities of ‘natural factories’ (living systems from which building blocks can be extracted). One such application where these ‘natural factories’ are exploited is in hybrid nanobiocomposites that blend favourable mechanical properties of biomolecules with well-characterized polymers. For example, defect-free nanocrystals of cellulose extracted from wood, tunicates and bacteria possess impressive mechanical properties such as an elastic modulus close to that of Kevlar [82] . New nanobiocomposites that incorporate CNCs, chitin [83] and other biological filler materials with impressive mechanical properties have recently been developed, and the resulting composites have shown enhanced elastic properties, thermal transitions (that is, glass transition temperature) and toughness. In addition, these materials have demonstrated some stimuli-responsive behaviours in which the elastic properties and specimen shape are greatly altered by varying moisture content [54] . These changes, also observed for amorphous cellulose, are the result of complex networks formed among biological filler particles that are disrupted by water molecules. This illustrates a key feature of this hybrid approach, in that it preserves key features and properties of the biological building blocks in a useful material form (that is, embedded in a well-known and characterized polymer). An additional design approach, biomimicry or biomimetic design, involves direct implementation of biological mechanisms and design principles in artificial systems and was pioneered by the Wright brothers when they modelled their first aircrafts based on their observations of birds in flight. As mentioned previously, recent mechanics research has demonstrated how the natural brick-and-mortar structures of nacre [7] , [52] and bone [84] , [85] are responsible for their high strength and toughness due to disparate material phases and geometrical arrangement and organizations [85] , [86] , [87] . Using this universal guiding principle, scientists have been able to create synthetic materials with poly(methyl methacrylate) and aluminium oxide to achieve ultra-high toughness with no biological components [6] , [38] , [88] through a programmed brick-and-mortar microstructure that helps to arrest crack propagation in the material, leading to increased strength and failure strains. Implementation of synthetic biomechanical designs through these manufacturing techniques has much potential in many areas of research, and, in particular, for improving temporal and spatial control of therapeutics, which could be informed by natural molecular mechanofunctionality in the body. Through mimicking the mechanical stimuli-responsive function of platelets for changing shape in response to high shear control, a recent approach aims to treat obstructed blood vessels through shear-controlled release of nanotherapeutics ( Fig. 5a ) [89] . The approach used intravenously injected microscale aggregates constructed from smaller therapeutic nanoparticles ( Fig. 5b ). The aggregates travelled through the bloodstream under normal shear conditions (below ∼ 70 dyne cm −2 ) until they were mechanically cued to dissemble in constricted blood flow, where shear may increase two orders of magnitude to over 1,000 dyne cm −2 . To ensure accurate triggering, rheology and fluid-material methods ( Fig. 5c ) were used to design the aggregate structure to remain stable during non-constricted circulation, but dissemble when subjected to sufficient hydrodynamic shear stress. This approach is potentially robust to error, because the release is triggered by environmental mechanical cues caused by targeted illness, rather than less direct molecular cues that may vary between tissues and patients. Furthermore, the mechanical release point could be tailored to individuals if necessary. 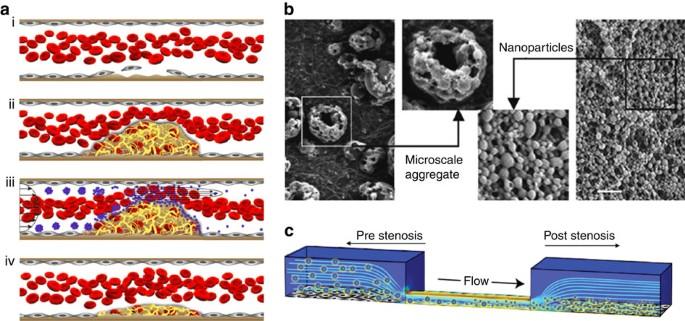Figure 5: Aggregated nanoparticles for mechanically responsive drug release through constricted blood flow89. (a) Experimental strategy schematic of (i) flowing red blood cells; (ii) being obstructed by growth of a thrombus obstruction; (iii) shear-activated nanotherapeutics (blue) dissociating near the thrombus via increased pressure from decreased blood vessel volume; and dissociated nanoparticles binding to the clot have progressively dissolved the obstruction (iv). (b) Shear-activated nanotherapeutics at the microscale (∼2 to 5 μm; left panel) are aggregates of poly (lactic-co-glycolic acid) nanoparticles (∼180 nm; right panel). (c) A microfluidic model that demonstrates how microscale aggregates break up when transitioning from the pre-stenosis region through constricted pathways where pressure is increased, eventually accumulating in endothelial cells along the bottom of the channel. Images are reproduced and adapted, with permission, from ref.89(copyright 2015, AAAS). Figure 5: Aggregated nanoparticles for mechanically responsive drug release through constricted blood flow [89] . ( a ) Experimental strategy schematic of (i) flowing red blood cells; (ii) being obstructed by growth of a thrombus obstruction; (iii) shear-activated nanotherapeutics (blue) dissociating near the thrombus via increased pressure from decreased blood vessel volume; and dissociated nanoparticles binding to the clot have progressively dissolved the obstruction (iv). ( b ) Shear-activated nanotherapeutics at the microscale ( ∼ 2 to 5 μm; left panel) are aggregates of poly (lactic-co-glycolic acid) nanoparticles ( ∼ 180 nm; right panel). ( c ) A microfluidic model that demonstrates how microscale aggregates break up when transitioning from the pre-stenosis region through constricted pathways where pressure is increased, eventually accumulating in endothelial cells along the bottom of the channel. Images are reproduced and adapted, with permission, from ref. 89 (copyright 2015, AAAS). Full size image Other drug delivery applications use strategies that require optimization of carrier shape, based on the many mechanical trade-offs that influence a particle’s in vivo journey [90] . Recent approaches have addressed this problem with synthetic molecules resembling red blood cells [91] and platelets [5] , thus providing a malleable shape for adhesion/elasticity and traversal through tight capillaries via elastic deformation. However, synthetic approaches could also leverage smart materials for reversible particle mechanics, when responding to stimuli such as light, pH and electrical fields [92] . With this approach, adaptive particles could embody an optimal travelling conformation, and then alter their shape via location-specific stimuli upon arrival. Drug release could be facilitated through the same principles present in self-cleaning biomimetic approaches [93] , and the materials of Fig. 4 provide many options for technological embodiment, thus leading to diverse design strategies for efficient and timely delivery of medicines. Box 2: Design approaches for mechanically passive and active muscle-based systems. Artificial muscle-based systems are drivers for many potential applications, including lab-on-chip actuation, robotic prosthetics and human tissue restoration—all of which have differing engineering needs and requirements. A recent synthetic muscle-manufacturing approach produced a passive actuation mechanism through braiding 32 two-ply, coiled, 102-μm-diameter muscle fibres manufactured from monofilament sewing thread [60] (panel a below). Particular benefits of this approach are the resulting muscle’s low cost, speed, scalability and nonhysteretic properties; the muscle can lift loads over 100 times greater than that of human muscle of the same length and weight. Its actuations result from the coiled structure of the muscle, which operate on principles of thermal expansion. Depending on the twist direction, it can contract or expand with heat. Passive approaches benefit from requiring no energy expenditure to contract, but are limited because of their dependence on external environmental cues. In contrast, active systems consume energy for quick and controlled responses, which are often necessary for organism survival and robotics applications. Active muscle functionality has been achieved in synthetic applications through the construction of an artificial jellyfish-like organism termed a medusoid [72] (panel b below). The medusoid consists of synthetic components with movement powered by biological muscle, transplanted from rat cardiac tissue that have larger fiber diameters in comparison with jellyfish muscle. Through this approach, the medusoid consistently swims via cyclical muscle contractions. These active muscle design principles can extend to systems where dynamic response is important, so that functionality can perpetuate regardless of fluctuating environmental conditions. Panel a is reproduced, with permission, from ref. 60 (copyright 2015, AAAS). Panel b is adapted from ref. 72 . Fundamental studies on mechanics in biology and their extension towards bio-inspired designs have set the stage for many promising future directions of engineering and scientific research. In particular, natural systems with mechanofunctionality can inform engineering endeavours far beyond simple material selection. Biological structures often reach high performance through system organization and interactions among materials across scales, as found in spider silk or stomatopod dactyl clubs. These mechanofunctional design principles can inform the design of synthetic systems, and many potential technologies could emerge that are inspired by natural passive and active actuation mechanisms and how they promote biological functions. Across many areas of potential applications, and medicine in particular, the need for dynamically responsive, multifunctional materials and stimuli-responsive systems could be met through bio-inspired approaches. To translate fundamental biological discoveries to engineered designs, an integrative viewpoint of length and timescales in responsive systems is needed, with considerations ranging from plants reconfiguring their structures based on environmental changes, to drug delivery mechanisms operating via mechanochemical cues. In particular, synthetic actuation mechanisms independent of specific chemical pathways, and instead based on concepts of scale, structure and geometry have the potential to enjoy wide-spread reception in engineered designs. Passively responsive systems capitalizing on anisotropy at both material and structure length scales are finding use in areas such as architecture, where wooden elements are used to open and close in response to humidity fluctuations to achieve building-scale homeostasis [94] . At smaller scales, active biomimetic materials could be used in artificial cells for in vivo travel to targeted sites for drug administration in a non-invasive manner [95] . Many challenges lie ahead in transferring mechanisms observed in nature to fully engineered systems. Most notably, many ideas are specific to material domains and length and timescales that cannot be synthetically replicated precisely, and rather require consideration of capturing the principles of a design. For example, in mimicking nacre or bone, not only is the brick-and-mortar geometry universally important, but also the relative stiffness of the two constituent phases; both of these strategies are representative of general design principles that could inform many engineered systems regardless of the material being used. In addition, the hierarchical complexity and functional disorder in biological materials calls for a shift in traditional preferences of designing single-scale, highly ordered systems. If these organizational considerations of natural systems are ignored, advances in the engineering of nanobiocomposites that utilize nanoblocks directly obtained from nature may fall short of reproducing and surpassing the impressive mechanical properties of natural materials in a scalable fashion [96] , [97] . Advances through recombinant techniques provide a systematic way of discerning emergent properties of natural building blocks in distinct material phases that could assist the transfer of natural principles to synthetic designs. A recombinant approach allows for the rearrangement/reshaping of naturally occurring building blocks that evolved in unrelated contexts (for example, elastin/resilin blends) to achieve unforeseen mechanical functionalities. Recombinant techniques eliminate the complexities of direct biomimicry, and hypothesis testing of structure–property relationships, especially when synthesis is combined with mechanical cues that mimic biological processes. Extending these studies to resolve size effects and interfacial mechanics of multiphasic systems could lead to new insights of how complex hierarchies and biological structures/chemistries affect emergent properties and functionalities relating to mechanics. Even with this knowledge, understanding how hybrid systems that interface biological building blocks with synthetic building blocks in non-obvious environments remains a challenge. Further research is necessary to optimize the resulting recombinant and composite materials for mechanofunctional biosystems, and is an important step in creating, for example, composites with increased toughness, tissues with increased elasticity/wear properties or structures that mimic the behaviour of natural systems. Beyond understanding the role of mechanics in natural systems, learning from these systems presents numerous opportunities for implementing findings in engineered designs using synthetic approaches. Specifically, these implementations are observable when comparing engineering metrics such as fracture toughness across scales in natural [98] , [99] , [100] , [101] , [102] , [103] , [104] , [105] and synthetic [106] , [107] , [108] systems, as we demonstrate in Fig. 6 . Here, the fracture toughness is defined as the energy required to fracture the system/material per unit area (J m −2 ) when considering relevant length scales. 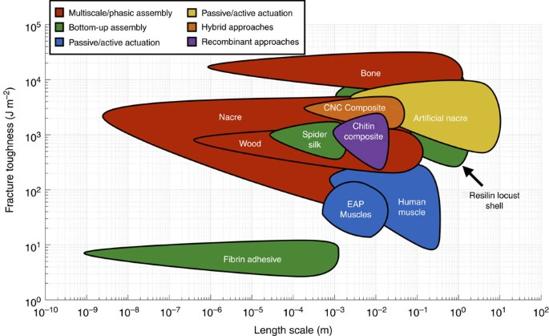Figure 6: Natural and synthetic approaches for meeting fracture toughness requirements at multiple scales. Systems are mapped according to the fracture toughness they achieve at varied length scales relevant to their spatial organization. Categories are differentiated based on approaches used in the mechanical fabrication of the systems, such as bone101, nacre98and wood100emerging naturally through multiscale/multiphasic organizations and spider silk105, fibrin adhesives104and resilin-based locust shells102emerging through bottom-up assembly processes. Systems with actuating functionality include EAP muscle’s99passive actuation and human muscle’s103active actuation. Artificial nacre106, chitin composites108and CNC composites107are representative of synthetic system approaches for biomimetic, recombinant and hybrid design strategies, respectively. Figure 6: Natural and synthetic approaches for meeting fracture toughness requirements at multiple scales. Systems are mapped according to the fracture toughness they achieve at varied length scales relevant to their spatial organization. Categories are differentiated based on approaches used in the mechanical fabrication of the systems, such as bone [101] , nacre [98] and wood [100] emerging naturally through multiscale/multiphasic organizations and spider silk [105] , fibrin adhesives [104] and resilin-based locust shells [102] emerging through bottom-up assembly processes. Systems with actuating functionality include EAP muscle’s [99] passive actuation and human muscle’s [103] active actuation. Artificial nacre [106] , chitin composites [108] and CNC composites [107] are representative of synthetic system approaches for biomimetic, recombinant and hybrid design strategies, respectively. Full size image When examining the systems shown in Fig. 6 , there is a diversity of performance for natural and synthetic systems with a multitude of strategies for achieving fracture toughness that could inform bio-inspired approaches. These strategies include multiscale organization as found in bone [101] , nacre [98] and wood [100] and systems constructed from the bottom-up to leverage emergent properties based on nanoscale characteristics (for example, polypetides in Fig. 2 ) such as spider silk [105] , fibrin adhesive [104] and locust shells [102] . These systems serve to inform engineering endeavours developed using biomimetic, hybrid and recombinant design approaches that mimic or surpass natural systems in their functionality and performance. There is still much research required for engineered systems to match natural system performance, such as artificial nacre [106] only achieving similar fracture toughness at higher length scales when compared with natural nacre. In some cases, however, engineered technologies closely match the performance of their biological analogues: electroactive polymer muscles [99] serve as an interesting passive alternative to active biological muscle [103] that achieve similar fracture toughness at a given length scale. Therefore, engineers can differentiate between these systems based on further criteria specific to a particular design scenario, which provides a greater number of feasible designs to explore in constructing mechanofunctional systems. The ability to understand how biological systems achieve beneficial functions through material designs and organizations can open many new routes in creating effective mechanofunctional technologies for diverse applications. Moreover, lessons learned from biology and biological systems are giving rise to applications beyond our own physiology and the medical field, where mechanical approaches to biological understanding and intervention have often been linked. The central role of mechanics in these systems will assist in developing novel engineering applications ranging from mechanically responsive synthetic muscle, to building better mechanical materials with functional silk, to creating stimuli-activated drug delivery systems—the areas where mechanics and biology intersect are numerous. Success in bringing experimental and computational approaches to bear with intricate mechanical and biological underpinnings will open a world of opportunities for fundamental scientific discoveries, while also leading the way towards ingenious and well-designed biomimetic technologies of the future. How to cite this article: Egan, P. et al . The role of mechanics in biological and bio-inspired systems. Nat. Commun. 6:7418 doi: 10.1038/ncomms8418 (2015).